ATG5 is induced by DNA-damaging agents and promotes mitotic catastrophe independent of autophagy Anticancer drug therapy activates both molecular cell death and autophagy pathways. Here we show that even sublethal concentrations of DNA-damaging drugs, such as etoposide and cisplatin, induce the expression of autophagy-related protein 5 (ATG5), which is both necessary and sufficient for the subsequent induction of mitotic catastrophe. We demonstrate that ATG5 translocates to the nucleus, where it physically interacts with survivin in response to DNA-damaging agents both in vitro and in carcinoma tissues obtained from patients who had undergone radiotherapy and/or chemotherapy. As a consequence, elements of the chromosomal passenger complex are displaced during mitosis, resulting in chromosome misalignment and segregation defects. Pharmacological inhibition of autophagy does not prevent ATG5-dependent mitotic catastrophe, but shifts the balance to an early caspase-dependent cell death. Our data suggest a dual role for ATG5 in response to drug-induced DNA damage, where it acts in two signalling pathways in two distinct cellular compartments, the cytosol and the nucleus. Macroautophagy (herein autophagy) is a process that occurs in response to stress in yeast, plants and mammalian cells by which a portion of the cytosol is sequestered in characteristic double- or multi-membrane vesicles to form autophagosomes. The molecular mechanisms of autophagosome formation are conserved in evolution and depend upon several autophagy-related proteins (ATGs). One of these is the ATG5, which conjugates with ATG12 to generate an E3 ubiquitin ligase-like enzyme required for autophagy [1] . Mice deficient in the atg5 gene die on the first day after birth [2] . Once formed, autophagosomes merge with lysosomes to form autolysosomes whose contents are degraded by lysosomal hydrolases [1] . Both autophagic and apoptotic pathways are activated during anticancer drug treatment [3] . As autophagy is a survival mechanism, one can speculate that autophagy induced by anticancer drugs might contribute to resistance to treatment in cancer patients [4] . The goal of our study was to investigate the role of ATG5 in the responses of cells to different DNA-damaging or antimitotic drugs at sublethal concentrations, which elicit little cell death. This allows dissecting in detail the biochemical responses to such an insult within the first days after treatment. We show that ATG5 is upregulated in cancer cells following treatment with DNA-damaging drugs, both under in vitro and in vivo conditions. Moreover, ATG5 also translocates to the nucleus where it physically associates with survivin. Mitotic catastrophe ensues, which, if the cytoplasmic autophagic pathway is concurrently blocked pharmacologically, proceeds rapidly to caspase-dependent cell death. DNA-damaging drugs induce ATG5 and mitotic catastrophe To investigate the role of autophagy in anticancer drug treatment, we decided to study the effects of different drugs at sublethal concentrations as determined for six antimitotic and DNA-damaging drugs in multiple experiments (the procedure is illustrated in Supplementary Fig. S1 ). Jurkat T cells were examined over the first 4 days after treatment with these six different drugs, each at the defined sublethal concentration, and classified morphologically as normal, apoptotic or abnormal. The latter case comprised enlarged cells with enlarged, irregular nuclei, cells exhibiting abnormal, multipolar mitoses and multinucleated cells ( Fig. 1a ). The apoptotic fraction was relatively modest at 2–6% ( Fig. 1a ). Cells treated with etoposide, cisplatin, taxol or nocodazole, however, showed 40–80% abnormal morphology, exhibiting enlarged, irregular nuclei, multipolar mitoses, or multiple nuclei, characteristic of mitotic catastrophe [5] . Mitotic catastrophe is defined in international consensus as an oncosuppressive phenomenon occurring during or after defective mitosis leading to death or senescence. [6] On the other hand, inefficient mitotic catastrophe with mitotic slippage can lead to the emergence of genetically unstable, tumorigenic, aneuploid cell population [5] , [6] , [7] . 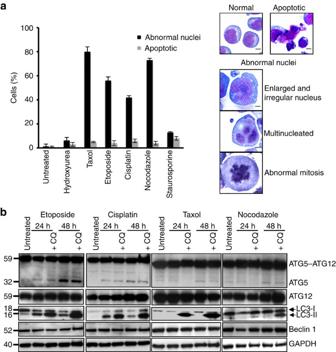Figure 1: Sublethal concentrations of anticancer drugs induce multinucleated cells and autophagy. (a) Morphological analysis. Jurkat T cells were cultured in the presence and absence of the indicated anticancer drugs for 48 h. Drug-treated cells were classified as normal, apoptotic or abnormal, with enlarged and irregular nuclei, with multipolar mitoses or multinucleated. Cultures treated with etoposide (0.25 μM), cisplatin (3 μM), taxol (4 nM) and nocodazole (10 nM) exhibited high levels of cells with abnormal nuclei. None of the treated populations showed a significant fraction of apoptosis (see alsoSupplementary Fig. S1). Values are means±s.d. for three independent experiments. Right: representative examples of these morphological categories are shown. Scale bar, 10 μM. Similar abnormalities were also seen after treating NB4 and MDA-MA-231 cells with etoposide or cisplatin (Supplementary Fig. S2). (b) Immunoblotting. Jurkat T cells were treated as indicated and ATG5 (monomeric and ATG12-conjugated), ATG12 (conjugated with ATG5), LC3 (18 and 16 kDa), Beclin 1 and GAPDH detected. Chloroquine (CQ) was employed to block lysosomal proteases. Each immunoblot is representative of at least three independent experiments. The same assays were performed using NB4 and MDA-MA-231 cells (Supplementary Fig. S2). Moreover, as a marker for autophagy onset, increased LC3-II formation following etoposide or cisplatin treatment was also documented using fluorescence microscopy (Supplementary Fig. S2). Full-length immunoblots are provided inSupplementary Fig. S8. Figure 1: Sublethal concentrations of anticancer drugs induce multinucleated cells and autophagy. ( a ) Morphological analysis. Jurkat T cells were cultured in the presence and absence of the indicated anticancer drugs for 48 h. Drug-treated cells were classified as normal, apoptotic or abnormal, with enlarged and irregular nuclei, with multipolar mitoses or multinucleated. Cultures treated with etoposide (0.25 μM), cisplatin (3 μM), taxol (4 nM) and nocodazole (10 nM) exhibited high levels of cells with abnormal nuclei. None of the treated populations showed a significant fraction of apoptosis (see also Supplementary Fig. S1 ). Values are means±s.d. for three independent experiments. Right: representative examples of these morphological categories are shown. Scale bar, 10 μM. Similar abnormalities were also seen after treating NB4 and MDA-MA-231 cells with etoposide or cisplatin ( Supplementary Fig. S2 ). ( b ) Immunoblotting. Jurkat T cells were treated as indicated and ATG5 (monomeric and ATG12-conjugated), ATG12 (conjugated with ATG5), LC3 (18 and 16 kDa), Beclin 1 and GAPDH detected. Chloroquine (CQ) was employed to block lysosomal proteases. Each immunoblot is representative of at least three independent experiments. The same assays were performed using NB4 and MDA-MA-231 cells ( Supplementary Fig. S2 ). Moreover, as a marker for autophagy onset, increased LC3-II formation following etoposide or cisplatin treatment was also documented using fluorescence microscopy ( Supplementary Fig. S2 ). Full-length immunoblots are provided in Supplementary Fig. S8 . Full size image As, under the conditions used, only little cell death occurred up to 4 days after initiation of treatment ( Supplementary Fig. S1 ), we investigated the molecular pathway of autophagy following exposure of Jurkat T cells to etoposide, cisplatin, taxol or nocodazole. Whereas etoposide and cisplatin induced autophagy as assessed with a biochemical analysis in which we observed the conversion from cytosolic LC3-I to membrane-bound LC3-II, these changes were largely absent in cells treated with taxol or nocodazole ( Fig. 1b ). A chloroquine control indicated that the accumulation of LC3-II after etoposide or cisplatin treatment was indeed a result of increased autophagic flux [8] . We then analysed ATG5, Beclin 1 (ATG6) and ATG12 expression levels. Autophagy induction was accompanied by increased levels of ATG5, which was largely seen as the ATG5–ATG12 conjugate (59 kDa), but also, although less, as the monomer (32 kDa) ( Fig. 1b ). The presence of ATG12 in the conjugate was confirmed with anti-ATG12 antibody ( Fig. 1b ). In contrast to ATG5, Beclin 1 was not induced by etoposide or cisplatin ( Fig. 1b ), and neither ATG5 nor Beclin 1 was significantly increased following taxol or nocodazole treatment ( Fig. 1b ). We subsequently investigated other cell types, observing a similar induction of autophagy associated with increases in ATG5 expression following etoposide or cisplatin treatment ( Supplementary Fig. S2a ). In these experiments, we confirmed the increased autophagic flux by demonstrating diminished levels of p62, a marker protein that functions as a link between LC3 and the ubiquitinated substrates [8] . Autophagosome formation could also be directly visualized when HeLa cells expressing fluorescent LC3 (LC3–GFP) were examined following etoposide or cisplatin exposure ( Supplementary Fig. S2b ). Moreover, treated cells showed characteristic mitotic catastrophe with enlarged, irregular nuclei and/or multiple nuclei after Giemsa/May–Grünwald staining ( Supplementary Fig. S2c ). Mitoses of HeLa cells expressing histone 2b (H2B–mCherry) and α-tubulin (EGFP–α-tubulin) [9] were photographed with fluorescence live microscopy after treatment with DNA-damaging drugs. Unlike the normal metaphase plate and bipolar spindles seen with untreated cells, drug-treated cells revealed the formation of multipolar spindles as well as misaligned and missegregated chromosomes characteristic of mitotic catastrophe [10] ( Fig. 2a ). Quantitative analysis of this cell population showed that the development of abnormal nuclei is time-dependent and occurs in the majority of both etoposide- and cisplatin-treated cells ( Fig. 2b ). Taken together, our findings indicate that both etoposide and cisplatin induce ATG5 expression, autophagy and mitotic catastrophe in multiple cell lines. In contrast, taxol and nocodazole treatment resulted in mitotic catastrophe, but without producing elevated ATG5 levels or increased autophagic activity. 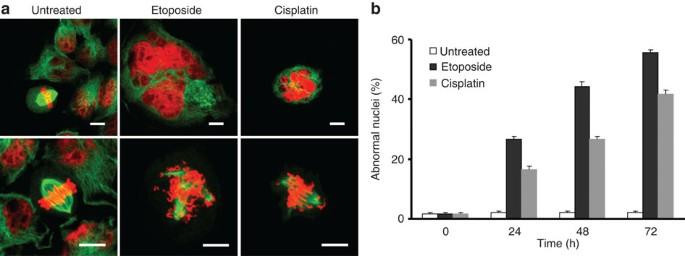Figure 2: DNA-damaging drugs induce mitotic catastrophe. (a) Time-lapse microscopy. HeLa H2B–mCherry–α-tubulin–EGFP cells were cultured in the presence and absence of etoposide and cisplatin, respectively. Treated cells frequently developed multiple nuclei, including micronuclei (upper panel), and demonstrated evidence of multipolar spindles and misaligned chromosomes (lower panel). Cells were also much larger than untreated cells (see alsoSupplementary Fig. S3). Scale bar, 10 μm. (b) Statistical analysis of the data shown above. At least 100 cells were counted for each drug exposure time according to the classification used inFig. 1. Values are means±s.d. (n=3). Figure 2: DNA-damaging drugs induce mitotic catastrophe. ( a ) Time-lapse microscopy. HeLa H2B–mCherry–α-tubulin–EGFP cells were cultured in the presence and absence of etoposide and cisplatin, respectively. Treated cells frequently developed multiple nuclei, including micronuclei (upper panel), and demonstrated evidence of multipolar spindles and misaligned chromosomes (lower panel). Cells were also much larger than untreated cells (see also Supplementary Fig. S3 ). Scale bar, 10 μm. ( b ) Statistical analysis of the data shown above. At least 100 cells were counted for each drug exposure time according to the classification used in Fig. 1 . Values are means±s.d. ( n =3). Full size image Critical role of ATG5 for mitotic catastrophe The elevation of ATG5 levels after etoposide and cisplatin treatment could be inhibited using two different short hairpin RNAs (shRNAs; Fig. 3a ). Blocking ATG5 expression prevented both the induction of autophagy, as assessed by LC3 immunoblotting ( Fig. 3a ), and the appearance of cells with abnormal nuclei ( Fig. 3b ). A control shRNA had no effect in these assays ( Fig. 3a,b ). These data suggested that increased levels of ATG5 are necessary for mitotic catastrophe following exposure to DNA-damaging drugs. 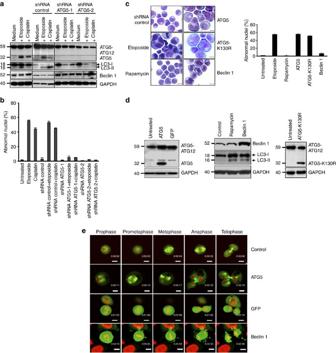Figure 3: ATG5 is necessary and sufficient for anticancer drug-induced mitotic catastrophe. (a) Immunoblotting. Jurkat T cells were cultured as indicated for 48 h. Only under conditions of ATG5 induction was evidence of increased autophagic activity obtained. Monomeric ATG5 (shown under the dotted line) was detected after a longer exposure time compared with the ATG5 conjugated with ATG12. Results are representative of three independent experiments. (b) Morphological analysis. Jurkat T cells were cultured as ina. Values are means±s.d. of three independent experiments. (c) Morphological analysis. Jurkat T cells were treated with the indicated drugs or transduced with lentivirus ATG5, ATG5-K130R, Beclin 1 or control constructs for 48 h. Enlarged and multinucleated cells were seen as a consequence of ATG5 or ATG5-K130R lentiviral gene transfer or of etoposide treatment. Increased Beclin 1 levels or rapamycin treatment had no such effect. Representative examples of morphology are shown. Scale bar, 10 μm. Right: statistical analysis of the data. At least 100 cells were counted for each condition. Values are means±s.d. (n=3). (d) Immunoblotting. Enforced expression of ATG5, Beclin 1, or ATG5-K130R following lentiviral gene transfer. (e) Time-lapse microscopy. HeLa H2B–mCherry–α-tubulin–EGFP cells were transduced by lentiviral gene transfer as indicated. Only ATG5-overexpressing cells demonstrated evidence for mitotic catastrophe (see alsoSupplementary Movies). As with the GFP control, the Beclin 1 construct also included GFP, hence the intensity in green was very high. Scale bar, 10 μm. Figure 3: ATG5 is necessary and sufficient for anticancer drug-induced mitotic catastrophe. ( a ) Immunoblotting. Jurkat T cells were cultured as indicated for 48 h. Only under conditions of ATG5 induction was evidence of increased autophagic activity obtained. Monomeric ATG5 (shown under the dotted line) was detected after a longer exposure time compared with the ATG5 conjugated with ATG12. Results are representative of three independent experiments. ( b ) Morphological analysis. Jurkat T cells were cultured as in a . Values are means±s.d. of three independent experiments. ( c ) Morphological analysis. Jurkat T cells were treated with the indicated drugs or transduced with lentivirus ATG5, ATG5-K130R, Beclin 1 or control constructs for 48 h. Enlarged and multinucleated cells were seen as a consequence of ATG5 or ATG5-K130R lentiviral gene transfer or of etoposide treatment. Increased Beclin 1 levels or rapamycin treatment had no such effect. Representative examples of morphology are shown. Scale bar, 10 μm. Right: statistical analysis of the data. At least 100 cells were counted for each condition. Values are means±s.d. ( n =3). ( d ) Immunoblotting. Enforced expression of ATG5, Beclin 1, or ATG5-K130R following lentiviral gene transfer. ( e ) Time-lapse microscopy. HeLa H2B–mCherry–α-tubulin–EGFP cells were transduced by lentiviral gene transfer as indicated. Only ATG5-overexpressing cells demonstrated evidence for mitotic catastrophe (see also Supplementary Movies ). As with the GFP control, the Beclin 1 construct also included GFP, hence the intensity in green was very high. Scale bar, 10 μm. Full size image To test whether ATG5 is sufficient to induce mitotic catastrophe, a human ATG5 construct was introduced into Jurkat T cells using a lentiviral gene expression system. As controls, Beclin 1 overexpression with a parallel construct or a drug treatment with rapamycin, both known to induce autophagy [11] , [12] , as well as etoposide treatment, were employed. Ectopic ATG5 overexpression, such as etoposide treatment, but neither Beclin 1 overexpression nor rapamycin treatment, resulted in multinucleated cells and mitotic catastrophe ( Fig. 3c , micrographs). Quantitative analysis revealed that more than 50% of the cells after lentiviral ATG5 gene transfer demonstrated abnormal nuclei ( Fig. 3c , right panel). The induction of autophagy by enforced Beclin 1 expression or rapamycin treatment was controlled by LC3 immunoblotting experiments ( Fig. 3d ). To answer the question whether ATG5 conjugation to ATG12 is required for induction of mitotic catastrophe, as is the case for inducing autophagy [13] , we also included cultures transduced with the mutant ATG5 (ATG5-K130R) ( Fig. 3c ), which is unable to conjugate with ATG12 (ref. 14 ). Interestingly, overexpression of ATG5-K130R also triggered the appearance of multinucleated cells ( Fig. 3c ), indicating that ATG5 is able to induce mitotic catastrophe independent of its conjugation with ATG12. Successful gene transfer was controlled by immunoblotting ( Fig. 3d ). Enforced ATG5 expression was employed in HeLa H2B–mCherry–α-tubulin–EGFP cells, which were then analysed by fluorescence live microscopy to show the morphology of the mitosis induced. Whereas uninfected cells or cells overexpressing green fluorescent protein (GFP) or Beclin 1 underwent mainly normal mitosis, cells overexpressing ATG5 exhibited unequally segregated chromosomes resulting in progeny with multiple nuclei ( Fig. 3e and Supplementary Movies 1–4 ). Moreover, the average time period between nuclear envelope breakdown and anaphase was longer in ATG5-overexpressing cells ( Supplementary Movies 1–4 ; control, 41 min; ATG5, 83 min; GFP, 42 min; Beclin 1, 43 min). The chromosomal abnormalities were visible already in the prometaphase and developed into nuclei that were irregular, shrunken and fragmented ( Fig. 3e and Supplementary Movie 2 ). Quantitative analysis revealed that the majority of abnormalities were seen in the anaphase, reaching ~50% of all mitotic cells observed in cytospin samples taken at 48 h after ATG5 transduction. An abnormal metaphase was seen in about 8% of cells undergoing mitosis at this time point. Moreover, ATG5-overexpressing cells exhibited a larger size (see also Supplementary Fig. S3 ) with rounded morphology ( Fig. 3e and Supplementary Movie 2 ). We next investigated whether enforced ATG5 expression would alter cell cycle regulation. Jurkat T cells were transduced with ATG5 or GFP, after which cell cycle analysis was performed daily using propidium iodide (PI) cytometry. Although GFP overexpression had only marginal effects, enforced expression of ATG5 resulted in an increased fraction of cells in the G2 or M phases of cell cycle, a fraction increasing with time of exposure ( Fig. 4a ). As a positive control, we used etoposide, which also induced such arrest ( Fig. 4a ). Interestingly, etoposide-mediated effects on the cell cycle appeared to depend on increased expression of ATG5, as shRNA ATG5 prevented accumulation of cells in G2 or M phases ( Fig. 4b ). To limit the number of different conditions to be analysed per experiment, in all subsequent assays, we have used etoposide as a model drug for inducing DNA damage. 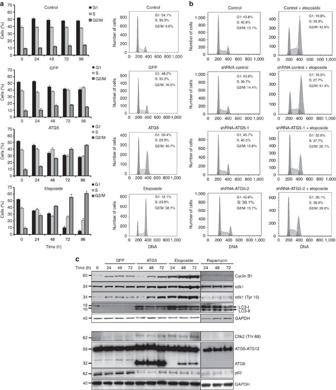Figure 4: Enforced expression of ATG5 induces G2- or M-phase arrest. (a) Cell cycle analysis. After lentivirus gene transfer, Jurkat T cells overexpressing ATG5 or GFP were followed for the indicated times and analysed for DNA content by flow cytometry. Untransduced cells were left untreated or treated with etoposide for comparison. Values are means±s.d. (n=3). Right: representative flow cytometry diagrams for the 48 h time point. (b) Cell cycle analysis. Jurkat cells were cultured as indicated for 48 h. Only under conditions of ATG5 induction, we observed an accumulation of cells in G2- or M-phase arrest. Results are representative of three independent experiments. (c) Immunoblotting. Jurkat T cells overexpressing ATG5 or GFP were cultured for the indicated times after transduction and analysed. As controls, cells were treated with etoposide or rapamycin. Although rapamycin, similar to etoposide, induced autophagy, no increase in ATG5 expression and no cell cycle arrest were observed. ATG5 overexpression and etoposide treatment resulted in a similar expression pattern for all proteins investigated. Each immunoblot is representative of at least three independent experiments. Figure 4: Enforced expression of ATG5 induces G2- or M-phase arrest. ( a ) Cell cycle analysis. After lentivirus gene transfer, Jurkat T cells overexpressing ATG5 or GFP were followed for the indicated times and analysed for DNA content by flow cytometry. Untransduced cells were left untreated or treated with etoposide for comparison. Values are means±s.d. ( n =3). Right: representative flow cytometry diagrams for the 48 h time point. ( b ) Cell cycle analysis. Jurkat cells were cultured as indicated for 48 h. Only under conditions of ATG5 induction, we observed an accumulation of cells in G2- or M-phase arrest. Results are representative of three independent experiments. ( c ) Immunoblotting. Jurkat T cells overexpressing ATG5 or GFP were cultured for the indicated times after transduction and analysed. As controls, cells were treated with etoposide or rapamycin. Although rapamycin, similar to etoposide, induced autophagy, no increase in ATG5 expression and no cell cycle arrest were observed. ATG5 overexpression and etoposide treatment resulted in a similar expression pattern for all proteins investigated. Each immunoblot is representative of at least three independent experiments. Full size image Protein levels of cell cycle regulators were studied to better understand the G2/M block. Unsurprisingly, cyclin B1 was stabilized by both etoposide treatment and ectopic ATG5 expression ( Fig. 4c , upper panel) in agreement with the increasing number of cells showing arrest at G2 or M phases [15] . Cyclin-dependent kinase 1 (cdk1) expression was somewhat increased and was found to be strongly phosphorylated in tyrosine 15 ( Fig. 4c , upper panel). In contrast, in GFP vector control or rapamycin-treated cells, tyrosine 15 phosphorylation of cdk1 was reduced ( Fig. 4c , upper panel). Both enforced expression of ATG5 and etoposide treatment led to phosphorylation of the Chk2 in threonine 68, thus activating the Chk2 signalling pathway ( Fig. 4c , lower panel). Moreover, these data clearly indicate that at least a cell subpopulation already exhibits an arrest in the G2 phase under these conditions. Moreover, lentiviral ATG5 gene transfer led to immediate conversion of cytosolic LC3-I into the autophagosome-specific LC3-II form, as did etoposide or rapamycin treatment ( Fig. 4c , upper panel). The degradation of p62 protein confirmed high autophagic activity in ATG5-overexpressing, as well as in etoposide- or rapamycin-treated, cells ( Fig. 4c , lower panel). We also analysed phosphorylated histone H2AX (phospho-H2AX) expression, an early DNA damage response marker [16] , by flow cytometry, confocal microscopy and immunoblotting. In contrast to untreated and ATG5- or GFP-overexpressing cells, this measure of DNA damage was only significantly elevated in cells treated with sublethal concentrations of etoposide ( Fig. 5a–c ). Moreover, we detected phospho-ataxia telangiectasia-mutated kinase (ATM) (Ser1981) and phospho-ataxia telangiectasia and Rad3-related kinase (ATR) (Ser428), two additional markers of the DNA damage response, and observed again no increased phosphorylation as a consequence of ATG5 gene transfer ( Fig. 5c ). 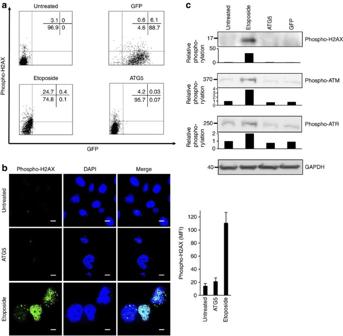Figure 5: Ectopic ATG5 expression does not induce DNA damage. (a) Flow cytometry. Untreated Jurkat T cells, cells treated with etoposide continuously (0.25 μM), or transduced with lentivirus ATG5 or GFP were cultured for 48 h, fixed, permeabilized and exposed to antiphospho-H2AX (Ser139) antibody, then stained with antimouse-APC-conjugated antibody, and analysed using a flow cytometer. (b) Confocal microscopy. Untreated HeLa cells, cells treated with etoposide continuously (0.25 μM), or transduced with lentivirus ATG5 were cultured for 48 h. Additional DAPI nuclear staining was used. Scale bar, 10 μm. Right: phospho-H2AX was quantified by measuring the mean fluorescence intensity (MFI) in five high-power fields of each condition using IMARIS software. Values are means±s.d. (c) Jurkat T cells were treated as inaand analysed by immunoblotting. Besides phospho-H2AX (Ser139), we also detected phospho-ATM (Ser1981) and phospho- ATR (Ser428), two additional markers of DNA damage response. Intensity of the protein bands were quantified with a Licor/Odyssey scanner and software (shown beneath each immunoblot). The fold change in phosphorylation levels compared with no treatment (untreated) are presented. The data in all panels are representative of at least three independent experiments. Full-length immunoblots are provided inSupplementary Fig. S9. Figure 5: Ectopic ATG5 expression does not induce DNA damage. ( a ) Flow cytometry. Untreated Jurkat T cells, cells treated with etoposide continuously (0.25 μM), or transduced with lentivirus ATG5 or GFP were cultured for 48 h, fixed, permeabilized and exposed to antiphospho-H2AX (Ser139) antibody, then stained with antimouse-APC-conjugated antibody, and analysed using a flow cytometer. ( b ) Confocal microscopy. Untreated HeLa cells, cells treated with etoposide continuously (0.25 μM), or transduced with lentivirus ATG5 were cultured for 48 h. Additional DAPI nuclear staining was used. Scale bar, 10 μm. Right: phospho-H2AX was quantified by measuring the mean fluorescence intensity (MFI) in five high-power fields of each condition using IMARIS software. Values are means±s.d. ( c ) Jurkat T cells were treated as in a and analysed by immunoblotting. Besides phospho-H2AX (Ser139), we also detected phospho-ATM (Ser1981) and phospho- ATR (Ser428), two additional markers of DNA damage response. Intensity of the protein bands were quantified with a Licor/Odyssey scanner and software (shown beneath each immunoblot). The fold change in phosphorylation levels compared with no treatment (untreated) are presented. The data in all panels are representative of at least three independent experiments. Full-length immunoblots are provided in Supplementary Fig. S9 . Full size image ATG5-mediated mitotic catastrophe is autophagy-independent As the ATG5-K130R mutant, which is itself unable to conjugate with ATG12, still induced mitotic catastrophe ( Fig. 3c ), we investigated the relationship between autophagy, G2 and M phase arrest, and mitotic catastrophe in more detail. Autophagy was induced both by starvation and by ectopic expression of Beclin 1. Although starvation indeed rapidly increased autophagic activity as assessed by accumulation of LC3-II and degradation of p62, no G2- and M-phase arrest was observed ( Supplementary Fig. S4a ). In fact, increased numbers of cells were observed in G1 arrest following starvation. Furthermore, cyclin B1 expression declined ( Supplementary Fig. S4a,b ). Similarly, overexpression of Beclin 1 was associated with induction of autophagy and reduced cyclin B1 levels, but had no effect on the cell cycle ( Supplementary Fig. S4a,b ). Moreover, neither starvation nor Beclin 1 transduction induced the morphological features of mitotic catastrophe ( Supplementary Fig. S4c ). Although this experiment confirmed that autophagy is not necessarily linked to G2- and M-phase arrest and mitotic catastrophe, an ATG5-mediated, increased autophagic activity might still be causally related to cell cycle arrest and mitotic catastrophe. Pharmacological inhibition of autophagy using 3-methyladenine (3-MA) (refs 17 , 18 ) blocked ATG5-mediated LC3-II accumulation and p62 degradation ( Fig. 6a ), demonstrating the functionality of the inhibitor in this system. However, 3-MA neither prevented ATG5-induced G2- and M-phase arrest ( Fig. 6b ) nor the nuclear abnormalities described above ( Fig. 6c ). 3-MA alone had no effect either on cell cycle or the fraction of cells with nuclear abnormalities. 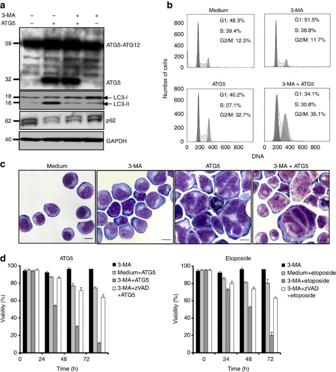Figure 6: Pharmacological inhibition of autophagy leads to a caspase-dependent cell death. (a) Immunoblotting. Jurkat T cells overexpressing ATG5 or control cells were cultured in the presence and absence of 3-MA for 48 h. 3-MA blocked the formation of LC3-II and p62 degradation, indicating that it indeed inhibited ATG5-induced autophagy. Results are representative of three independent experiments. (b) Cell cycle analysis. Normal Jurkat T cells and cells overexpressing ATG5 were cultured for 48 h in the presence and absence of 3-MA. Induction of G2- or M-phase arrest was seen as a consequence of ATG5 overexpression independent of treatment with 3-MA, as normal Jurkat T cells exhibited no G2/M arrest following 3-MA treatment. Representative flow cytometry diagrams are shown (n=3). Moreover, induction of autophagy by Beclin 1 overexpression or starvation failed to produce cell cycle arrest (Supplementary Fig. S4). (c) Morphological analysis. Normal Jurkat T cells and cells overexpressing ATG5 were cultured for 48 h in the presence and absence of 3-MA and analysed. Representative examples of morphology are shown (n=3); large multinucleated cells and cells with abnormal nuclei were seen as a consequence of ATG5 overexpression independent of 3-MA. Neither induction of autophagy by Beclin 1 overexpression nor starvation resulted in such abnormal cells (Supplementary Fig. S4). Scale bar, 10 μm. (d) Viability assays. Jurkat T cells either overexpressing ATG5 following lentiviral gene transfer or treated with etoposide were cultured in the presence and absence of the indicated pharmacological inhibitors for the indicated times to block autophagy and caspase activity. All values are means±s.d. (n=3). Figure 6: Pharmacological inhibition of autophagy leads to a caspase-dependent cell death. ( a ) Immunoblotting. Jurkat T cells overexpressing ATG5 or control cells were cultured in the presence and absence of 3-MA for 48 h. 3-MA blocked the formation of LC3-II and p62 degradation, indicating that it indeed inhibited ATG5-induced autophagy. Results are representative of three independent experiments. ( b ) Cell cycle analysis. Normal Jurkat T cells and cells overexpressing ATG5 were cultured for 48 h in the presence and absence of 3-MA. Induction of G2- or M-phase arrest was seen as a consequence of ATG5 overexpression independent of treatment with 3-MA, as normal Jurkat T cells exhibited no G2/M arrest following 3-MA treatment. Representative flow cytometry diagrams are shown ( n =3). Moreover, induction of autophagy by Beclin 1 overexpression or starvation failed to produce cell cycle arrest ( Supplementary Fig. S4 ). ( c ) Morphological analysis. Normal Jurkat T cells and cells overexpressing ATG5 were cultured for 48 h in the presence and absence of 3-MA and analysed. Representative examples of morphology are shown ( n =3); large multinucleated cells and cells with abnormal nuclei were seen as a consequence of ATG5 overexpression independent of 3-MA. Neither induction of autophagy by Beclin 1 overexpression nor starvation resulted in such abnormal cells ( Supplementary Fig. S4 ). Scale bar, 10 μm. ( d ) Viability assays. Jurkat T cells either overexpressing ATG5 following lentiviral gene transfer or treated with etoposide were cultured in the presence and absence of the indicated pharmacological inhibitors for the indicated times to block autophagy and caspase activity. All values are means±s.d. ( n =3). Full size image ATG5- or etoposide-driven mitotic catastrophe was associated with little cell death; however, in combination with 3-MA treatment we observed dramatic cell death, which could be blocked by pharmacological inactivation of caspases using 20 μM zVAD (z-Val-Ala-Asp) treatment ( Fig. 6d ). Thus, ATG5 induces G2- and M-phase arrest and mitotic catastrophe independently of its capacity to enhance autophagic activity. Autophagy, on the other hand, is required for cell survival under these conditions. ATG5 translocates to the nucleus We hypothesized that if increased ATG5 expression after etoposide or cisplatin treatment is indeed functionally linked to G2- and M-phase arrest and mitotic catastrophe, it may require translocation to the nucleus to fulfill this role. Indeed, as could be demonstrated with cell fractionation experiments, etoposide treatment caused increased, especially monomeric ATG5 levels in both cytoplasm and nucleus of Jurkat T cells ( Fig. 7a ). The purity of cytoplasmic and nuclear fractions was controlled here using antibodies against caspase-3 and lamin B, which served as markers for the cytoplasmic and nuclear compartments, respectively ( Fig. 7a ). 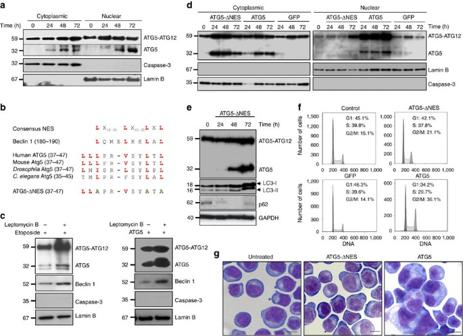Figure 7: Translocation of ATG5 is required for cell cycle arrest and mitotic catastrophe. (a) Subcellular fractionation and immunoblotting. Jurkat T cells were cultured in the presence of etoposide for the indicated times. Following etoposide treatment, the ATG5 monomer was newly present in both cytoplasm and nucleus. The exposure of the ATG5 monomer (shown under the dotted line) was longer than that shown above for the ATG5 conjugated to ATG12. Full-length immunoblots are provided inSupplementary Fig. S10. (b) A comparison of ATG5 sequences in different species demonstrates the presence of a conserved putative NES, similar to that present in Beclin 1. The sequence alignment was performed with Clustal W using sequence data obtained from GenBank. The characteristic leucines are indicated in red and the resulting sequence of ATG5-ΔNES, following mutation of three leucines within this motif, is shown. (c) Subcellular fractionation and immunoblotting of the nuclear fraction. Jurkat T cells, either treated with etoposide, or overexpressing ATG5 following lentiviral gene transfer, were cultured in the presence and absence of leptomycin B for 72 h. Leptomycin B increased relative ATG5 and Beclin 1 levels in the nucleus. (d) Subcellular fractionation and immunoblotting. Jurkat T cells were transduced to express ATG5-ΔNES, ATG5, or GFP. Although increased levels of ATG5 were observed in both cytoplasm and nucleus, ATG5-ΔNES accumulated following lentiviral gene transfer in the cytoplasm only. Full-length immunoblots are provided inSupplementary Fig. S11. (e) Immunoblotting. ATG5-ΔNES overexpression induced LC3-II formation and p62 degradation, indicating increased autophagic flux. (f) Cell cycle analysis. Jurkat T cells overexpressing ATG5 or ATG5-ΔNES, as well as control cells were cultured for 48 h. Induction of G2 and M phase arrest was seen as a consequence of ATG5, but not ATG5-ΔNES overexpression. As an additional control, we transduced cells with GFP, which, similar to ATG5-ΔNES-overexpressing cells, failed to exhibit G2- and M-phase arrest. Representative flow cytometry diagrams are shown (n=3). (g) Morphological analysis. Non-transduced Jurkat T cells and cells overexpressing ATG5 or ATG5-ΔNES were cultured for 48 h. Large, multinucleated cells were seen as a consequence of ATG5, but not ATG5-ΔNES overexpression. Representative examples are shown (n=3). Scale bar, 10 μm. Figure 7: Translocation of ATG5 is required for cell cycle arrest and mitotic catastrophe. ( a ) Subcellular fractionation and immunoblotting. Jurkat T cells were cultured in the presence of etoposide for the indicated times. Following etoposide treatment, the ATG5 monomer was newly present in both cytoplasm and nucleus. The exposure of the ATG5 monomer (shown under the dotted line) was longer than that shown above for the ATG5 conjugated to ATG12. Full-length immunoblots are provided in Supplementary Fig. S10 . ( b ) A comparison of ATG5 sequences in different species demonstrates the presence of a conserved putative NES, similar to that present in Beclin 1. The sequence alignment was performed with Clustal W using sequence data obtained from GenBank. The characteristic leucines are indicated in red and the resulting sequence of ATG5-ΔNES, following mutation of three leucines within this motif, is shown. ( c ) Subcellular fractionation and immunoblotting of the nuclear fraction. Jurkat T cells, either treated with etoposide, or overexpressing ATG5 following lentiviral gene transfer, were cultured in the presence and absence of leptomycin B for 72 h. Leptomycin B increased relative ATG5 and Beclin 1 levels in the nucleus. ( d ) Subcellular fractionation and immunoblotting. Jurkat T cells were transduced to express ATG5-ΔNES, ATG5, or GFP. Although increased levels of ATG5 were observed in both cytoplasm and nucleus, ATG5-ΔNES accumulated following lentiviral gene transfer in the cytoplasm only. Full-length immunoblots are provided in Supplementary Fig. S11 . ( e ) Immunoblotting. ATG5-ΔNES overexpression induced LC3-II formation and p62 degradation, indicating increased autophagic flux. ( f ) Cell cycle analysis. Jurkat T cells overexpressing ATG5 or ATG5-ΔNES, as well as control cells were cultured for 48 h. Induction of G2 and M phase arrest was seen as a consequence of ATG5, but not ATG5-ΔNES overexpression. As an additional control, we transduced cells with GFP, which, similar to ATG5-ΔNES-overexpressing cells, failed to exhibit G2- and M-phase arrest. Representative flow cytometry diagrams are shown ( n =3). ( g ) Morphological analysis. Non-transduced Jurkat T cells and cells overexpressing ATG5 or ATG5-ΔNES were cultured for 48 h. Large, multinucleated cells were seen as a consequence of ATG5, but not ATG5-ΔNES overexpression. Representative examples are shown ( n =3). Scale bar, 10 μm. Full size image We detected in ATG5 a conserved sequence homologous to the leucine-rich nuclear export signal (NES) of Beclin 1 (ref. 19 ; Fig. 7b ). Exposure of etoposide-treated or ATG5-overexpressing cells to leptomycin B, an inhibitor of the exportin-1 (CRM1)-dependent nuclear export [20] , caused accumulation of both Beclin 1 and ATG5 in the nucleus ( Fig. 7c ). We prepared a mutated ATG5 construct in which the human ATG5 sequence was modified, replacing three of the four most conserved leucines with alanines ( Fig. 7b ). Surprisingly, expression of this NES-mutated form of ATG5 (ATG5-ΔNES) failed to accumulate in the nucleus and was detectable in the cytoplasm only ( Fig. 7d ), where it was still able to induce autophagy as assessed by LC3-II accumulation and p62 degradation ( Fig. 7e ). In contrast to ATG5, however, enforced expression of this ATG5-ΔNES caused neither G2 and M phase arrest ( Fig. 7f ) nor mitotic catastrophe ( Fig. 7g ). These findings suggest that the putative NES must overlap a cryptic, but functional nuclear localization motif (NLS) required for the transport of ATG5 from the cytoplasm to the nucleus. ATG5 and survivin physically interact in the nucleus We hypothesized that increased nuclear expression of ATG5 might disturb chromosome segregation by interacting with other proteins, such as elements of the chromosomal passenger complex contributing to chromatin-associated spindle formation [21] . Interestingly, we could show that following enforced ATG5 expression, survivin was upregulated, specifically in the mRNA levels of the so-called wild-type survivin [22] , whereas the expression levels of other survivin isoforms did not change ( Supplementary Fig. S5 ). To test the possibility that survivin interacts physically with ATG5 following etoposide treatment or ectopic overexpression, we performed coimmunoprecipitation assays using antibodies for both ATG5 and survivin. The presence of survivin in the ATG5 immunoprecipitate and, reciprocally, ATG5 in the survivin immunoprecipitate, was unambiguous both with ATG5 overexpression and etoposide treatment of Jurkat T cells ( Fig. 8a ). In a further coimmunoprecipitation experiment, we demonstrated that ATG5-ΔNES failed to interact with survivin ( Fig. 8b ), suggesting that the interaction takes place in the nucleus, where ATG5-ΔNES is absent, or, alternatively, that an interaction with survivin depends on the mutated leucine-rich sequence modified in ATG5-ΔNES. In contrast to ATG5-ΔNES, the ATG5-K130R mutant, which is able to mediate mitotic catastrophe ( Fig. 3c ), interacted with survivin ( Fig. 8c ). Moreover, calpain-mediated 24-kDa truncated ATG5 (ref. 23 ) was unable to interact with survivin ( Fig. 8d ), suggesting that the amino-terminal part of ATG5 is most likely not responsible for the interaction with survivin. 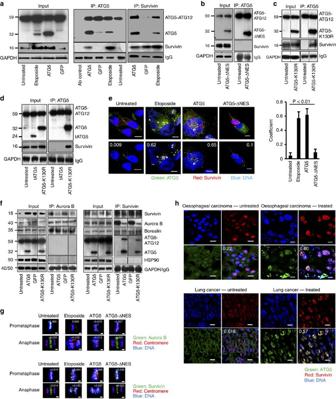Figure 8: Nuclear ATG5 physically interacts with survivin. (a) Lysates of Jurkat T cells overexpressing ATG5 or treated with etoposide (48-h cultures) were immunoprecipitated with anti-ATG5 or antisurvivin antibodies. A physical interaction between ATG5 and survivin, absent in untreated or GFP-expressing control cells, was detected reciprocally. Full-length immunoblots are provided inSupplementary Fig. S12. (b) Jurkat T cells overexpressing ATG5-ΔNES exhibited no ATG5/survivin molecular interaction. (c) The ATG5-K130R mutant did show coprecipitation of survivin with ATG5. (d) Calpain-mediated, truncated ATG5 (tATG5), that is, the N-terminal part of ATG5, failed to bind survivin. The ATG5-K130R mutant was the control. (e) Confocal microscopy. MDA-MA-231 cells were etoposide treated or transduced as indicated (48-h cultures) and stained. In untreated cells, survivin and ATG5 were in the cytosol with no colocalization. ATG5-transduced cells exhibited ATG5/survivin colocalization in the nucleus. ATG5-ΔNES-transduced cells showed survivin, but not ATG5, in the nuclei of cycling cells. Numerical analysis was performed and Pearson’s correlation coefficients are indicated in the images. Scale bar, 10 μm. Right: Statistical analysis (analysis of variance) is presented in which the results of ten representative cells within each group were integrated. Values are means±s.d. (f) The physical interaction between Aurora B and survivin was analysed reciprocally and reduced in cells expressing high levels of nuclear ATG5. Neither ATG5 nor HSP90 were detectable in the Aurora B-containing immune precipitate, but ATG5 molecularly interacted with survivin. Results representative of three independent experiments. (g) Confocal microscopy. HeLa cells treated with etoposide or transduced as indicated (48-h cultures) were stained with centromere-specific antiserum and anti-Aurora B (top panels) or antisurvivin antibodies (lower panels). In untreated or ATG5-ΔNES transduced cells, both Aurora B and survivin were recruited to prometaphase centromeres and located at the central spindle during anaphase where they no longer colocalized with centromeres. In contrast, etoposide-treated or ATG5-transduced cells recruited much less Aurora B to prometaphase centromeres. Such recruitment, however, was observed during anaphase. Compared with cells in normal mitosis, survivin, although reduced, was recruited to centromeres in prometaphase, but, similar to Aurora B, remained attached to centromeres during anaphase. Such mislocation of Aurora B and survivin was associated with severe chromosome alignment and segregation defects. Colocalization images were prepared using Imaris software. Numerical analysis was performed and correlation coefficients are indicated. Scale bar, 2 μm. (h) Confocal microscopy. Sections of lung (non-small-cell lung cancer) and oesophageal carcinoma stained for ATG5 and survivin expression. In untreated patients, ATG5 expression in cancer cells was slight and mainly cytosolic. Following radio- and/or chemotherapy, ATG5 was preferentially expressed in the nucleus and colocalized with survivin. Overlay images present the average Pearson’s correlation coefficient as calculated with Imaris. Results are representative of three independent experiments. Scale bar, 10 μm. Figure 8: Nuclear ATG5 physically interacts with survivin. ( a ) Lysates of Jurkat T cells overexpressing ATG5 or treated with etoposide (48-h cultures) were immunoprecipitated with anti-ATG5 or antisurvivin antibodies. A physical interaction between ATG5 and survivin, absent in untreated or GFP-expressing control cells, was detected reciprocally. Full-length immunoblots are provided in Supplementary Fig. S12 . ( b ) Jurkat T cells overexpressing ATG5-ΔNES exhibited no ATG5/survivin molecular interaction. ( c ) The ATG5-K130R mutant did show coprecipitation of survivin with ATG5. ( d ) Calpain-mediated, truncated ATG5 (tATG5), that is, the N-terminal part of ATG5, failed to bind survivin. The ATG5-K130R mutant was the control. ( e ) Confocal microscopy. MDA-MA-231 cells were etoposide treated or transduced as indicated (48-h cultures) and stained. In untreated cells, survivin and ATG5 were in the cytosol with no colocalization. ATG5-transduced cells exhibited ATG5/survivin colocalization in the nucleus. ATG5-ΔNES-transduced cells showed survivin, but not ATG5, in the nuclei of cycling cells. Numerical analysis was performed and Pearson’s correlation coefficients are indicated in the images. Scale bar, 10 μm. Right: Statistical analysis (analysis of variance) is presented in which the results of ten representative cells within each group were integrated. Values are means±s.d. ( f ) The physical interaction between Aurora B and survivin was analysed reciprocally and reduced in cells expressing high levels of nuclear ATG5. Neither ATG5 nor HSP90 were detectable in the Aurora B-containing immune precipitate, but ATG5 molecularly interacted with survivin. Results representative of three independent experiments. ( g ) Confocal microscopy. HeLa cells treated with etoposide or transduced as indicated (48-h cultures) were stained with centromere-specific antiserum and anti-Aurora B (top panels) or antisurvivin antibodies (lower panels). In untreated or ATG5-ΔNES transduced cells, both Aurora B and survivin were recruited to prometaphase centromeres and located at the central spindle during anaphase where they no longer colocalized with centromeres. In contrast, etoposide-treated or ATG5-transduced cells recruited much less Aurora B to prometaphase centromeres. Such recruitment, however, was observed during anaphase. Compared with cells in normal mitosis, survivin, although reduced, was recruited to centromeres in prometaphase, but, similar to Aurora B, remained attached to centromeres during anaphase. Such mislocation of Aurora B and survivin was associated with severe chromosome alignment and segregation defects. Colocalization images were prepared using Imaris software. Numerical analysis was performed and correlation coefficients are indicated. Scale bar, 2 μm. ( h ) Confocal microscopy. Sections of lung (non-small-cell lung cancer) and oesophageal carcinoma stained for ATG5 and survivin expression. In untreated patients, ATG5 expression in cancer cells was slight and mainly cytosolic. Following radio- and/or chemotherapy, ATG5 was preferentially expressed in the nucleus and colocalized with survivin. Overlay images present the average Pearson’s correlation coefficient as calculated with Imaris. Results are representative of three independent experiments. Scale bar, 10 μm. Full size image Evidence for molecular interactions between ATG5 and survivin was also obtained when cells were analysed by immunofluorescence staining and confocal microscopy, as performed with the large, flat cells of the MDA-MA-231 line. In untreated interphase cells, endogenous ATG5 and survivin were expressed in the cytosol, but no significant colocalization was observed ( Fig. 8e ). Upon etoposide treatment or ectopic ATG5 overexpression, significant levels of ATG5 were observed in the nucleus where colocalization with survivin could be detected ( Fig. 8e ). In contrast, in ATG5-ΔNES-overexpressing cells ATG5 expression was seen in the cytosol only, again with little evidence of colocalization with survivin ( Fig. 8e ). Aurora B is a protein that is known to interact with survivin in forming the chromosomal passenger complex [24] . We observed reduced levels of interaction between Aurora B and survivin in both Aurora B-specific and survivin-specific immunoprecipitates of cells overexpressing ATG5 ( Fig. 8f ). This finding is consistent with the hypothesis that ATG5 competes with Aurora B for available survivin, with the consequence, presumably, that formation of the chromosomal passenger complex is disturbed. The ATG5-K130R mutant had the same effect ( Fig. 8f ). Within the immunoprecipitate specific for Aurora B, ATG5 was not detectable ( Fig. 8f ). Moreover, the amount of borealin, another chromosomal passenger complex protein [25] , was unaffected by increased levels of nuclear ATG5 or ATG5-K130R ( Fig. 8f ). We also searched for HSP90 in this protein complex, as an earlier report suggested that survivin interacts with HSP90 to prevent proteasomal degradation of survivin [26] . We obtained, however, no evidence that HSP90 is physically linked to either Aurora B or survivin ( Fig. 8f ). We next analysed the recruitment of chromosomal passenger complex proteins to centromeres during mitosis [27] , [28] . Using indirect immunofluorescence experiments, we observed that during abnormal mitosis of etoposide-treated or ATG5-transduced cells, Aurora B appeared to be mislocated and was found much less at centromeres in prometaphase as compared with normal mitoses of untreated cells ( Fig. 8g ). ATG5-ΔNES-overexpressing cells demonstrated normal Aurora B recruitment to centromeres, suggesting that only the presence of newly recruited nuclear ATG5 is able to bring about the displacement of this chromosomal passenger protein. In contrast to Aurora B, survivin did not appear to be reduced or displaced from the centromeres at prometaphase in cells with increased levels of nuclear ATG5 ( Fig. 8g ). However, in contrast to normal mitoses in which survivin was located at the central spindle during anaphase, survivin was displaced and remained at the centromeres in the majority of mitotic etoposide-treated or ATG5-transduced cells ( Fig. 8g ). Similarly, Aurora B was also mislocated during anaphase in cells with elevated nuclear ATG5 levels and was not found at the central spindle as seen during normal mitoses in untreated or ATG5-ΔNES transduced cells ( Fig. 8g ). These abnormalities, seen in both prometaphase and anaphase were associated with severe chromosome alignment and segregation defects ( Fig. 8g ), supporting the assumption that the nuclear interaction between ATG5 and survivin is followed by a disturbance of the chromosomal passenger complex during mitosis. We have also observed nuclear ATG5 expression in carcinoma tissues of the lung and esophagus after patients had received DNA-damaging radio- and/or chemotherapy ( Fig. 8h ). In contrast, in specimens obtained from patients having received no prior radio- and/or chemotherapy, ATG5 was detected almost entirely in the cytosol ( Fig. 8h ). Moreover, cancer cells expressed survivin at high levels, which strongly colocalized with ATG5 after anticancer treatment ( Fig. 8h ). We also obtained evidence for reduced survivin–Aurora B molecular interactions in specimens of cancer cells having received treatment ( Supplementary Fig. S6 ). These data clearly suggest that the findings reported in this paper are of in vivo relevance. In this study we have investigated molecular events involved in mitotic catastrophe caused by DNA-damaging agents and report the following new findings: first, these agents upregulate ATG5 expression, which is both necessary and sufficient to induce mitotic catastrophe in an autophagy-independent manner. Second, ATG5 is not only a cytosolic protein, it is also expressed in the nucleus. Nuclear ATG5 accumulates following DNA damage, a finding, observed under both in vitro and in vivo conditions. Interestingly, a NES-like motif apparently overlaps with cryptic sequences acting as a NLS, thus supporting nuclear translocation. Third, ATG5 associates with survivin in the nucleus following drug-induced DNA damage under both in vitro and in vivo conditions. Fourth, ATG5 seems likely to influence the composition of the chromosomal passenger complex by reducing the interaction between survivin and Aurora B. Fifth, mitotic catastrophe induced by nuclear ATG5 is not associated with induction of cell death, as long as an autophagic response is maintained. Following a pharmacological block of autophagy, however, the cells promptly undergo caspase-dependent cell death. In agreement with earlier reports [3] , [5] , this study supports the idea that anticancer drugs cause apoptosis, autophagy and mitotic catastrophe. Whereas apoptosis of cancer cells is a clear therapeutic goal, the induction of both autophagy and mitotic catastrophe may cause problems. Autophagy can, at least under certain conditions, exhibit tumour-promoting effects [4] . Similarly, mitotic catastrophe does not always lead to cell death and has been described as a cancer cell survival mechanism [29] , [30] . Moreover, mitotic catastrophe in the absence of subsequent cell death favours potentially oncogenic polyploidization [6] . It should be noted that under the conditions used in this study, mitotic catastrophe, whether induced by anticancer drugs or by ectopic ATG5 overexpression, was generally not followed by cell death in the time frame investigated (up to 96 h for the in vitro studies). Interestingly, ATG5 appeared to have an important dual role in this scenario. Although cytosolic ATG5 contributed to increased autophagic activity, nuclear ATG5 induced mitotic catastrophe, which, however, did not immediately trigger cell death, as long as autophagy pathways were active. These data support the view that mitotic catastrophe is not per se a cell death mechanism [6] , [7] . Treatment of multiple cancer cell lines with etoposide or cisplatin resulted in increased ATG5 expression. Although the molecular mechanisms following DNA damage, particularly the transcriptional regulation of ATG5 gene expression, remain to be determined, we analysed the functional consequences of increased ATG5 expression following drug treatment. Using two different shRNA ATG5 approaches for blocking increased ATG5 expression, we demonstrated that elevated levels of ATG5 are necessary for both drug-induced autophagy and mitotic catastrophe. To show that ATG5 is sufficient for inducing the same effects, we overexpressed ATG5 in cancer cells. In agreement with earlier work [23] , enforced ATG5 expression resulted in increased levels of autophagy as assessed by LC3-II and p62 immunoblotting. Increased autophagic flux was additionally demonstrated by analysing the amount of LC3-II in the presence and absence of a lysosomal protease inhibitor. Moreover, besides induction of autophagy, we observed cell enlargement, aberrant nuclei, multinuclear cells and multipolar mitosis, suggesting that cells undergo mitotic catastrophe following both DNA-damaging drug treatment or ectopic ATG5 overexpression. Indeed, ATG5 overexpression itself, similar to etoposide and cisplatin treatment, resulted in Chk2 activation and inactivation of the cyclin B1/cdk1 complex, consistent with the induction of a G2 arrest [31] . The activation of Chk2 after ATG5 gene transfer suggested that ATG5 overexpression might have caused DNA damage, which could have activated the G2 checkpoint and explain the observed cell cycle arrest. However, immunoblots showed no evidence for increased phosphorylation of H2AX, ATM or ATR, three markers of the DNA damage response. Assessing phosphorylated H2AX by flow cytometry and confocal microscopy, we observed no or only very subtle DNA damage, which, however, is unlikely to explain the major mislocalization of survivin and Aurora B during mitosis. With our approach, quantitative data obtained with flow cytometry was based solely on DNA amount and failed to distinguish between G2 phase and M phase cells. On the basis of microscopic examination of stained cells and counts of 1,000 cells for each time point, the fraction of abnormal nuclei was 14% at 24 h after transfection, 45% at 48 h and 57% at 72 h. The fraction of cells in mitosis was relatively constant at 2.8–3.6%. These values correspond fairly well with the G2 phase plus M-phase fraction found with flow cytometry. We also studied the possible role of p53, which is required for induction of cell death following DNA damage [32] . Using p53-inducible Saos-2 cells, we obtained no evidence for a role of p53 in ATG5-mediated mitotic catastrophe ( Supplementary Fig. S7 ), a finding that is in agreement with another report [33] . On the other hand, it has been suggested that the final fate of cells suffering mitotic catastrophe may depend on the status of p53 (ref. 34 ). Thus, we must speculate that some activity of ATG5 leads to crosstalk with the DNA damage response pathway. The fact that autophagy protects cells from genotoxic stress and maintains genome integrity has already been established [35] . Autophagy, however, is unlikely to be itself responsible for the G2 arrest and mitotic catastrophe for the following reasons. First, autophagy induced by the overexpression of Beclin 1 or starvation did not lead to mitotic catastrophe. Second, 3-MA, an inhibitor of autophagy, did not block ATG5-mediated effects on cell cycle or mitotic catastrophe. Third, a mutant ATG5, unable to conjugate with ATG12 and incompetent to initiate autophagy, still induced G2 arrest and mitotic catastrophe. Together with earlier work [14] , [23] , these data suggest that ATG5 exerts alternative functions beyond and independent of autophagy. The nuclear localization of ATG5 was a surprising finding, observed not only in cell lines but also in the lung and oesophageal carcinoma tissues. But how can ATG5 translocate to the nucleus? We identified a conserved putative NES in ATG5 without, however, any canonical NLS [36] . This lack is not infrequent with proteins entering the nucleus [37] . HIV-1 vpr exhibits no canonical NLS, but carries an arginine-rich region, which overlaps with and influences recognition of the leucine-rich NES. This region is both a functional NLS and a NES, having a role in nuclear shuttling of protein and viral nucleocapsid at the time of initial infection [37] , [38] . We prepared mutants of the putative NES of ATG5, replacing three of the conserved leucines with alanines (ATG5-ΔNES). Following mutagenesis of conserved leucines in this sequence, we observed, not as expected, an increased accumulation of ATG5 in the nucleus owing to a failure of export, but rather, much like the pattern with vpr , the absence of ATG5 in the nucleus. Most interestingly, ATG5-ΔNES also fails to cause G2 arrest or mitotic catastrophe. Inhibition of the CRM1-dependent nuclear export following leptomycin B treatment of cells overexpressing wild-type ATG5 does lead to nuclear accumulation. Survivin protects cells from apoptosis both in vitro and in vivo by inhibiting the mitochondrion/caspase-9-activated ‘intrinsic’ pathway and is associated with an X-linked inhibitor of apoptosis protein [39] , [40] . Survivin also regulates cell division and participates in forming the chromosome passenger complex responsible for chromosome segregation [21] , [24] . Hence, survivin is expressed in the G2 phase of cell cycle [41] . It has also been shown that survivin is strongly expressed in most human cancers [42] . We demonstrate here that certain DNA-damaging drugs upregulate both ATG5 and survivin expression, which, subsequently, colocalize in the nucleus. Physical interaction between ATG5 and survivin was demonstrated by both immunoprecipitation experiments and confocal microscopy. Importantly, we also show here upregulation and colocalization of ATG5 and survivin, as well as evidence for reduced survivin–Aurora B molecular interactions under in vivo conditions using patient-derived cancer tissues. ATG5-ΔNES, unable to enter the nucleus, did not associate with survivin and did not induce a G2 arrest or abnormal mitosis. Thus, the association of ATG5 and survivin is consistent with the observed mitotic defects in metaphase, because survivin contributes to chromatin-associated spindle formation [21] . However, as shown in this report it is likely that this molecular interaction changes the composition of the chromosomal passenger complex, as the interaction between Aurora B and survivin was seen to be reduced. Moreover, we obtained evidence that both Aurora B and survivin were displaced in prometaphases and anaphases in cells undergoing abnormal mitosis after etoposide treatment or enforced ATG5 expression. These abnormalities were associated with a severe disturbance in chromosome alignment and segregation. In agreement with these findings, Aurora B mislocation had previously been reported to result in loss of chromosome alignment and disruption of cytokinesis in the absence of cell death [28] . Mitotic catastrophe has previously been observed in cells treated with small interfering RNA survivin [43] . Therefore, it is likely that nuclear ATG5 acts as a functional survivin antagonist leading to Aurora B mislocation during mitosis. These abnormalities, however, are also associated with the displacement of survivin itself, particularly during anaphase. Regardless of the exact molecular consequences of the ATG5/survivin molecular interactions, our data suggest that ATG5 interferes with the roles of survivin and Aurora B in chromosome alignment and segregation during mitosis. Thus, ATG5, similar to survivin, exhibits different roles in the cytosol and nucleus. The two different roles of ATG5 are of obvious medical importance in connection with anticancer therapy. Moreover, our data explain, at least partially, why autophagy can have tumour-promoting activities [4] . The fraction of cells that survive mitotic catastrophe is aneuploid, genetically highly diverse and, therefore, potentially very dangerous [6] , [7] . Inhibition of autophagy seems to be a reasonable therapeutic strategy to induce cell death under conditions of mitotic catastrophe. Reagents Rapamycin, hydroxyurea, nocodazole, staurosporine, taxol, PI, 3-MA, chloroquine and leptomycin B were purchased from Sigma-Aldrich (Buchs, Switzerland). Etoposide was from Bristol-Myers Squibb AG (Baar, Switzerland) and cisplatin from Nycomed Pharma AG (Dübendorf, Switzerland). If not otherwise indicated, etoposide was used at 0.25 μM and cisplatin at 3 μM. The caspase inhibitor zVAD-fluoromethylketone was obtained from BD Biosciences (Erembodegem, Belgium). DAPI (4′,6-diamidino-2-phenylindole) was from Invitrogen (Paisley, UK). Cells MDA-MA-231 and HeLa cells were obtained from the American Type Culture Collection (ATCC, Rockville, MD, USA). NB4 cells were from the Deutsche Sammlung von Mikroorganismen und Zellkulturen, GmbH (DSMZ, Braunschweig, Germany). Jurkat T cells (J16 clone) were the gift of Dr M. Peter (German Cancer Research Center, Heidelberg, Germany). HKF1-(HeLa Kyoto with FRT-site) H2B–mCherry–α-tubulin–EGFP cells were provided by Dr D.W. Gerlich (Institute of Biochemistry, ETH Zurich, Zurich, Switzerland) [9] . HeLa cells expressing GFP-LC3 were the gift of Dr T. Yoshimori, Osaka University, Osaka, Japan) [44] . Jurkat T and NB4 cells were grown in RPMI 1640 (Life Technologies) with 10% heat-inactivated FCS. HeLa and MDA-MA-231 cells were grown in DMEM supplemented with 5% heat-inactivated FCS. Tumour tissues Specimens were paraffin sections from surgical material of six oesophageal carcinoma and six non-small-cell lung cancer patients obtained from the archive of the histology laboratory of the Institute of Pathology, University of Bern. The study was approved by the internal review board of the University Hospital Bern. Patients were either untreated or had received several cycles of standard neoadjuvant chemotherapy (lung cancer patients: cisplatin and docetaxel [45] ) or combined radio- and chemotherapy (oesophagus patients: cisplatin and 5-fluorouracil [46] ). Site-directed mutagenesis The ATG5-ΔNES mutant lacking the NES was constructed essentially as described for Beclin 1 (ref. 19 ). Amino acid mutations on L39A, L45A and L47A were generated using QuickChange Site-Directed Mutagenesis Kit (Stratagene Europe, Amsterdam, The Netherlands) using the following primer sequences: forward, 5′-TAC TAT TTG CTT GCA CCA AGA GTA AGT TAT GCT ACG GCA GTA ACT GAC AAA-3′ and reverse, 5′-TTT GTC AGT TAC TGC CGT AGC ATA ACT TAC TGG TGC AAG CAA ATA GTA-3′. The ATG5-K130R mutant, unable to conjugate with ATG12, was generated as previously described [14] . The mutated ATG5 sequences were confirmed by sequence analysis. The constructs were subcloned into the pWPT vector. Lentiviral gene transfer and gene silencing Human ATG5 (Gene ID: 9474, NM_004849), ATG5-ΔNES, ATG5-K130R, calpain-mediated truncated ATG5 (ref. 4 ) and GFP were subcloned into the HIV-derived vector pWPT, containing a cytomegalovirus promoter [47] . Two types of shRNA ATG5 were used: ATG5-1 shRNA was subcloned in pMSCV-Puro-miR30 (ref. 48 ), which was the gift of Dr M. Narita (Cambridge Research Institute, Cambridge, UK), as well as ATG5-2 shRNA, which was in pLKO.1 and obtained from Sigma-Aldrich. Human Beclin 1 (Gene ID: 8678, NM_003766) was subcloned in a CAD vector containing GFP [49] , which was obtained from Dr M. Tschan (Department of Clinical Research, University of Bern, Bern, Switzerland). Recombinant virus constructs were produced by calcium phosphate transfection together with the envelope vector PMD2.G and the packaging vectors psPAX2 for lentivirus (all provided by Dr D. Trono, University of Geneva, Switzerland) into 293T cells. For virus stocks, the supernatant was collected 24, 48 and 72 h after transfection and cleared. Virus was immediately concentrated at 4 °C in a Beckman Coulter ultracentrifuge (Palo Alto, CA, USA) with the SW41-Ti rotor (RCF: 55,000 g for 90 min). Pellets were re-suspended in RPMI 1640 medium with 10% FCS in 1/10th the volume of the original culture supernatant. Concentrated virus was used at a multiplicity of infection of 25 as described [50] . The expression of transduced genes was controlled by immunoblotting. The efficacy of gene transfer was controlled by counting GFP-positive cells following pWPT-GFP transduction and was between 90 and 100%. Gel electrophoresis and immunoblotting Cells (0.5–1.0 × 10 6 ) were washed with Dulbecco’s PBS (DPBS), lysed with lysate buffer (50 mM Tris, pH 7.4, 150 mM NaCl, 10% glycerol, 1% Triton-X100, 2 mM EDTA, 10 mM Na 4 P 2 O 7 , 50 mM NaF, 200 μM Na 3 VO 4 ) or with 2 × SDS loading buffer, and cell lysates passed 10–15 times through a 26-gauge needle. Equal amounts of protein (30–50 μg per lane) of the cell lysates were loaded on NuPAGE gels (Invitrogen). Gels were electroblotted onto polyvinylidene difluoride membranes (Immobilion-P; Millipore). The blots were incubated with primary antibodies at 4 °C overnight in transfer buffer solution with 0.1% Tween-20 and 5% non-fat dry milk and developed with the ECL-technique (ECL-Kit, Amersham). Primary antibodies were purchased as follows: monoclonal antihuman ATG5 and anti-LC3 antibodies were from NanoTools (Taningen, Germany). Polyclonal rabbit, affinity-purified antiphospho-Chk2 (Thr68), antiphospho-cdk1 (Tyr15), anticaspase-3 and anti-Beclin 1, as well as monoclonal mouse anticyclin B1, rabbit antisurvivin, rabbit anti-Aurora B, rabbit anti-HSP-90 and rabbit antiphospho-ATR (Ser428) antibodies were obtained from Cell Signaling Technology (Danvers, MA, USA). Monoclonal antiphospho-H2AX (Ser139) and antiphospho-ATM (Ser1981) antibodies were from Upstate Cell Signaling Solutions (Lake Placid, NY, USA). Rabbit anti-p62 antibody was from Sigma-Aldrich and anti-ATG12 antibody from R&D Systems (Minneapolis, MN, USA). Monoclonal mouse antisurvivin and anti-cdk1, as well as polyclonal goat anti-lamin B and rabbit antiborealin antibodies were from Santa Cruz Biotechnology (Santa Cruz, CA, USA). All primary antibodies were used at 1:500 or 1:1,000 dilutions. Monoclonal anti-GAPDH antibody was from Chemicon International, Inc. (Temecula, MA, USA) and used at 1:5,000. Subcellular fractionation Jurkat T cells (10–30 × 10 6 ) were treated and genetically modified as indicated, cultured as indicated, then washed with cold PBS, resuspended in hypotonic lysis buffer (10 mM Hepes, pH 8, 5 mM KCl, 2 mM MgCl 2 , 2 mM DDT) and Dounce homogenized (10–15 strokes) on ice. To separate cytoplasmic (supernatant) and nuclear (pellet) fractions, the homogenate was centrifuged at 1,000 g for 5 min at 4 °C. The fractions were lysed by addition of 2 × SDS loading buffer, equal amounts of proteins were loaded on 12% NuPAGE gels, and subsequently transferred onto polyvinylidene difluoride membranes as described above. Caspase-3 and lamin B were used as markers to control the fractionation. Coimmunoprecipitation Jurkat T cells (1 × 10 7 ) were lysed in total lysate buffer (50 mM Tris, pH 7.4, 150 mM NaCl, 40 mM β-glycerol phosphate, 10 mM NaF, 0.5% (vol/vol) IGEPAL, 0.1% deoxycholate, 30 μg ml −1 RNase, 80 U ml −1 micrococcal nuclease (Sigma-Aldrich), 10 μm prefabloc, protease inhibitor cocktail tablets (Roche Diagnostics), 100 μM ATP, 100 μM MgCl 2 , 100 nM okadaic acid and 0.3 mM Na-vanadate). Lysates were passed 20–30 times through a 26-gauge needle, centrifuged and precleared by centrifugation after incubation at 4 °C with 10 μl of prewashed 50% Protein A/Protein G-agarose beads (Santa Cruz) for 1 h. Primary antibodies used were: rabbit polyclonal anti-ATG5 (2 μg), rabbit antisurvivin (2 μg), rabbit anti-Aurora B (2 μg) (all Cell Signaling Technology), or rabbit IgG control (2 μg) (Dako, Baar, Switzerland). Overnight incubation with primary antibodies was followed by a 2-h incubation at 4 °C with 30 μl of pre-washed 50% Protein A/Protein G-agarose beads. Immunocomplexes were washed four times with lysis buffer, denatured, loaded on a 12% NuPAGE gel and processed by immunoblotting as described above. Confocal laser-scanning microscopy Cells were grown on washed coverslips, fixed and permeabilized. Indirect immunostainings were performed at 4 °C overnight using the following primary antibodies: monoclonal anti-ATG5 (1/100; Nanotools), rabbit antisurvivin antibody (1/500; Cell Signaling Technology), rabbit anti-aurora B antibody (1/100; Cell Signaling Technology), centromere antiserum (1/800; Europa Bioproducts Ltd, Cambridge, UK) and monoclonal antiphospho-H2AX (1/1,000). Mouse and rabbit control antibodies were used at the same concentrations in each experiment. Incubation with appropriate Alexa Fluor 488 goat antimouse IgG and Alexa Fluor 532 goat antirabbit IgG (both Molecular Probes and Invitrogen), as well as APC donkey anti-mouse IgG (Jackson ImmunoResearch, West Baltimore Pike, PA, USA) was performed in the dark at room temperature for 1 h. The coverslips were mounted on slides using Prolong Gold containing DAPI (Invitrogen). The slides were analysed by confocal laser-scanning microscopy (LSM 5 Exciter microscope, Carl Zeiss, Jena, Germany). Expression of ATG5, survivin and Aurora B was also analysed in paraffin-embedded tissue specimens derived from surgical material of cancer patients by immunofluorescence [51] . For colocalization studies, unprocessed data sets were analysed using the Imaris software (Bitplane AG, Zurich, Switzerland), considering each single layer of a stack separately. Quantitative data for colocalization events were determined by the statistics modules in the colocalization and Voxelshop software of the Imaris package. Intensities were given as sum of all colocalizing voxels in a data set, and a computer image was generated. For quantitative analysis of colocalization, the Pearson’s correlation coefficient was calculated [52] . Time-lapse microscopy HeLa H2B–mCherry–α-tubulin–mEGFP cells were seeded on glass-bottomed tissue culture dishes (MatTek Corporation, Ashland, MA, USA) and transduced with lentiviral particles containing human full-length ATG5, human Beclin 1 or GFP. Time-lapse microscopy data were acquired using an Axio observer microscope (Carl Zeiss) equipped with a camera (Digital Pixel Imaging) and a full-enclosure environmental chamber heated to 37 °C with 5% CO2 and humidifier. Frames were recorded every 5 min for a total of 72 h ( Supplementary Movies 1–4 ). Fluorescence was visualized through an LSM 5 Exciter microscope (AOTF attenuation of 3%, laser lines 488 nM and 543 nM. Photomultiplier tube voltage was 802 V, amplifier offset −0.223) and acquisition was performed using a Plan-Apochromat objective ( × 63, numerical aperture 1.4, oil immersion) and a 270-μm confocal pinhole aperture. Time periods between nuclear envelope breakdown and anaphase were determined as previously reported [53] . Flow cytometry For cell cycle analysis, cells were treated and genetically modified as indicated, washed with DPBS containing 2% FCS, fixed with 70% ethanol at −20 °C for 1 h, pelleted, resuspended in DPBS and permeabilized with 0.125% Triton X-100. RNase (0.2 mg ml −1 ) was added and cells were stained with 40 μg ml −1 PI. Viability was assessed by exclusion of 1 μM ethidium bromide [23] , [54] , [55] . The expression of phosphorylated H2AX was measured following staining, which is described above (confocal microscopy). Cells were analysed by flow cytometry (FACS Calibur, BD Biosciences), and data processed by FlowJo software (Tree Star, Inc., Ashland, OR, USA). How to cite this article: Maskey, D. et al . ATG5 is induced by DNA-damaging agents and promotes mitotic catastrophe independent of autophagy. Nat. Commun. 4:2130 doi: 10.1038/ncomms3130 (2013).